Coherent optical wavelength conversion via cavity optomechanics Both classical and quantum systems utilize the interaction of light and matter across a wide range of energies. These systems are often not naturally compatible with one another and require a means of converting photons of dissimilar wavelengths to combine and exploit their different strengths. Here we theoretically propose and experimentally demonstrate coherent wavelength conversion of optical photons using photon–phonon translation in a cavity-optomechanical system. For an engineered silicon optomechanical crystal nanocavity supporting a 4-GHz localized phonon mode, optical signals in a 1.5 MHz bandwidth are coherently converted over a 11.2 THz frequency span between one cavity mode at wavelength 1,460 nm and a second cavity mode at 1,545 nm with a 93% internal (2% external) peak efficiency. The thermal- and quantum-limiting noise involved in the conversion process is also analysed, and in terms of an equivalent photon number signal level are found to correspond to an internal noise level of only 6 and 4 × 10 −3 quanta, respectively. The ability to coherently convert photons between disparate wavelengths has broad technological implications, not only for classical communication systems but also future quantum networks [1] , [2] , [3] . For example, hybrid quantum networks require a low loss interface capable of maintaining quantum coherence while connecting spatially separate systems operating at incompatible frequencies [4] . For this reason, photons operating in the low loss telecommunications band are often proposed as a conduit for connecting different physical quantum systems [5] . It has also been realized that a wide variety of quantum systems lend themselves to coupling with mechanical elements. A coherent interface between mechanics and optics, then, could provide the required quantum links of a hybrid quantum network [6] . Until now, most experiments demonstrating both classical and quantum wavelength conversion have utilized intrinsic optical nonlinearities of materials [7] , [8] , [9] , [10] , [11] , [12] . The nonlinear interaction of light with acoustic or molecular mechanical vibrations of materials, for instance, enables a great many optical functions used in high-speed optical communication systems today [8] . With the technological advancements in the fields of nanomechanics and nanophotonics, it is now possible to engineer interactions of light and mechanics. Progress in this area has included enhanced nonlinear optical interactions in structured silica fibres [13] , near quantum-limited detection of nanomechanical motion [14] , and the radiation pressure cooling of a mesoscopic mechanical resonator to its quantum ground state of motion [14] , [15] . Coupling of electromagnetic and mechanical degrees of freedom, in which the coherent interaction rate is larger than the thermal decoherence rate of the system, as realized in the ground-state cooling experiments, opens up an array of new applications in classical and quantum optics. This realization, along with the inherently broadband nature of radiation pressure, has spawned a variety of proposals for converting between photons of disparate frequencies [6] , [16] , [17] , [18] through interaction with a mechanical degree of freedom—proposals that are but one of many possible expressions of hybrid optomechanical systems [4] . Such cavity-optomechanical systems are not just limited to the optical frequency domain, but may also find application to the interconversion of microwave and optical photons [17] , [19] , enabling a quantum–optical interface to superconducting quantum circuits [20] . In this Article, we demonstrate optical wavelength conversion utilizing a simple hybrid optomechanical system consisting of an acoustic and optical resonator formed from the top silicon device layer of a silicon-on-insulator wafer typically used in the microelectronics industry. Through nanoscale lithographic patterning, an optomechanical crystal (OMC) resonator [21] is formed, which supports a 4-GHz mechanical resonance colocalized with two optical resonances in the S and C telecommunications bands. The extreme localization of both acoustic and optical energy in this OMC resonator results in a strong radiation pressure interaction between both optical modes and the mechanical motion of the resonator, enabling conversion of light between the two optical cavity modes, which span a frequency of 11.2 THz. Optical wavelength conversion is demonstrated over the 1.5 MHz bandwidth of the mechanical resonator at a peak internal efficiency exceeding 90% (the end-to-end measured efficiency is limited to 2% by the optical fibre coupling efficiency to the optical cavities), and with a thermal-limited noise of only 6 quanta, well above the quantum-limited noise of 4 × 10 −3 quanta. Theoretical description As illustrated in Fig. 1a , conceptually the proposed system for wavelength conversion may be thought of as consisting of two optical cavities coupled to the same mechanical resonator. 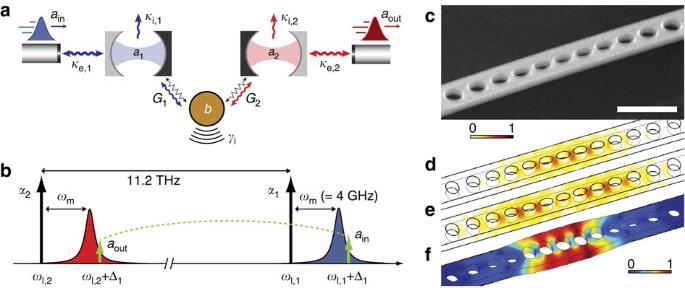Figure 1: System model and physical realization. (a) Diagram of the wavelength conversion process as realized via two separate Fabry–Perot cavities. The two optical cavity modes,a1anda2, are coupled to the same mechanical mode,b, with coupling strengthsG1andG2, respectively. The optical cavity modes are each coupled to an external waveguide (with coupling strengthsκe,1andκe,2), through which optical input and output signals are sent. The optical cavities also have parasitic (intrinsic) loss channels, labelledκi,1andκi,2, whereas the mechanical mode is coupled to its thermal bath at rateγi. (b) Schematic indicating the relevant optical frequencies involved in the wavelength conversion process. The cavity control laser beams, labelledα1andα2, are tuned to a mechanical frequency red of the corresponding optical cavity resonances. An input signal (ain) is sent into the input cavity at frequencyωl,1+Δ1. The input signal is converted into an output signal (aout) at frequencyωl,2+Δ1via the optomechanical interaction. (c) Scanning electron micrograph of the fabricated silicon nanobeam optomechanical cavity. Scale bar, 1 μm. (d,e) Finite element method (FEM) simulation of the electromagnetic energy density, normalized to the maximum modal energy, of the first- (d) and (e) second-order optical cavity modes of the silicon nanobeam. (f) FEM simulation of the displacement field of the colocalized mechanical mode, normalized to the maximum modal displacement. Figure 1: System model and physical realization. ( a ) Diagram of the wavelength conversion process as realized via two separate Fabry–Perot cavities. The two optical cavity modes, a 1 and a 2 , are coupled to the same mechanical mode, b , with coupling strengths G 1 and G 2 , respectively. The optical cavity modes are each coupled to an external waveguide (with coupling strengths κ e,1 and κ e,2 ), through which optical input and output signals are sent. The optical cavities also have parasitic (intrinsic) loss channels, labelled κ i,1 and κ i,2 , whereas the mechanical mode is coupled to its thermal bath at rate γ i . ( b ) Schematic indicating the relevant optical frequencies involved in the wavelength conversion process. The cavity control laser beams, labelled α 1 and α 2 , are tuned to a mechanical frequency red of the corresponding optical cavity resonances. An input signal ( a in ) is sent into the input cavity at frequency ω l,1 +Δ 1 . The input signal is converted into an output signal ( a out ) at frequency ω l,2 +Δ 1 via the optomechanical interaction. ( c ) Scanning electron micrograph of the fabricated silicon nanobeam optomechanical cavity. Scale bar, 1 μm. ( d , e ) Finite element method (FEM) simulation of the electromagnetic energy density, normalized to the maximum modal energy, of the first- ( d ) and ( e ) second-order optical cavity modes of the silicon nanobeam. ( f ) FEM simulation of the displacement field of the colocalized mechanical mode, normalized to the maximum modal displacement. Full size image Motion of the mechanical resonator induces a shift proportional to the amplitude of motion in the resonance frequency of each of the optical cavities, corresponding to the usual radiation pressure interaction in a cavity-optomechanical system. In this case, the two optical cavities are assumed to have different resonant frequencies, between which the desired optical wavelength conversion occurs. For each of the optical cavities, a pump laser beam red-detuned by the mechanical resonance frequency is used to couple the optical cavity modes to the mechanical resonator via the radiation pressure interaction, resulting in a coherent mixing of optical and mechanical degrees of freedom. Under these conditions, the shared mechanical resonator acts as a bridge between the two optical cavities, whereby incident optical radiation resonant with one optical mode is converted into mechanical motion, which is then converted back into optical radiation at the frequency of the other optical mode. This process, akin to the four-wave mixing found in coherent anti-Stokes Raman spectroscopy [22] , can result in near-unity conversion efficiency by both matching the pump-induced coupling rates of the mechanical mode to each of the optical cavity modes and increasing the optomechanical coupling rate above that of the intrinsic loss rate of the mechanical resonator. The interaction Hamiltonian describing the radiation pressure interaction between the two cavity modes and the mechanical resonator is given by , where â k ( ) are the annihilation operators for the optical cavity modes (common mechanical mode), and g k is the optomechanical coupling rate between the mechanical mode and the k th cavity mode ( k =1,2). Physically, g k represents the frequency shift of cavity mode k owing to the zero-point motion of the mechanical resonator. Wavelength conversion is driven by two control laser beams ( α k in Fig. 1b ), of frequency ω l, k and nominal detuning δ k ≡ ω k − ω l, k = ω m to the red of cavity resonance at frequency ω k . In the resolved sideband regime, where ω m ≫ K k ( κ k the bandwidth of the k th cavity mode), the spectral filtering of each cavity preferentially enhances photon–phonon exchange. The resulting beam-splitter-like Hamiltonian is (refs 17 , 23 ), where is the parametrically enhanced optomechanical coupling rate owing to the α k control beam ( n c, k is the control beam-induced intracavity photon number). In the weak-coupling limit, G k ≪ k k , this interaction effectively leads to an additional mechanical damping rate, . The degree to which this optomechanical loss rate dominates the intrinsic mechanical loss is called the cooperativity, C k = γ OM, k / γ i . At large cooperativities, the optomechanical damping has been used as a nearly noiseless loss channel to cool the mechanical mode to its ground state [14] , [15] . In the case of a single optical cavity system, it has also been used as a coherent channel allowing inter-conversion of photons and phonons leading to the observation of electromagnetically induced transparency (EIT) [24] , [25] . In the double optical cavity system presented here, coherent wavelength conversion of photons results. As shown in Fig. 1a , each optical cavity is coupled not just to a common mechanical mode, but also to an optical bath at rate κ i, k and to an external photonic waveguide at rate κ e, k (the total cavity linewidth is κ k = κ i, k + κ e, k ). The external waveguide coupling provides an optical interface to the wavelength converter, and in this work consists of a single-transverse-mode waveguide, bidirectionally coupled to each cavity mode. The efficiency of the input/output coupling is defined as η k = κ e, k /2 κ k , half that of the total bidirectional rate. Although the wavelength converter operates symmetrically, here we will designate the higher frequency cavity mode ( k =1) as the input cavity and the lower frequency cavity ( k =2) as the output cavity. As shown in Fig. 1b , photons sent into the wavelength converter with detuning Δ 1 ~ ω m from the control laser α 1 , are converted to photons Δ 1 detuned from the control laser α 2 , an 11.2 THz frequency span for the device studied here. The details of the conversion process can be understood by solving the Heisenberg–Langevin equations (see Supplementary Methods and refs 17 , 18 , 26 ). We linearize the system and work in the frequency domain, obtaining through some algebra the scattering matrix element s 21 ( ω ), which is the complex, frequency-dependent conversion coefficient between the input field at cavity â 1 and the output field at cavity â 2 . This coefficient is given by the expression where γ = γ i + γ OM,2 + γ OM,1 is the total mechanical damping rate and equal to the bandwidth of the conversion process. From this expression, the spectral density of a converted signal S out,2 ( ω ), given the input signal spectral density S in,1 ( ω ), may be found and is given by These spectral densities have units of photons per hertz per second and are proportional to optical power. The added noise, n added , arises from thermal fluctuations of the mechanical system and the quantum back-action noise of light present in each optical mode. From here, we see that in a system with ideal cavity–waveguide coupling, ( η 1 , η 2 =1), the peak internal photon conversion efficiency is given by This efficiency only depends on the internal coupling of the optomechanical system, and for both C 1 = C 2 and C 1 , C 2 ≫ 1, approaches unity. The latter condition can be understood from requiring the coupling between the optical and mechanical modes to overtake the intrinsic mechanical loss rate, while the first requirement is owing to impedance-like matching [17] . The total system efficiency is η max = η 1 η 2 η max,int . Device description and characterization The optomechanical system used in this work, shown in Fig. 1c–f , consists not of a separate set of optical cavities, but rather of a single OMC nanobeam cavity. The OMC nanobeam is fabricated from a silicon-on-insulator microchip [21] , in which the top, 220 nm thick, silicon device layer is patterned with a quasi-periodic linear array of etched air holes. The resulting silicon beam is 10 μm long and 600 nm wide. The hole radii and positions are designed by numerical optimization and repeated simulations, as discussed in detail in [27] . The larger air holes on either end of the beam induce Bragg-like reflection of both guided optical and acoustic waves, resulting in strongly confined optical and mechanical resonances at the beam’s centre. The device used in this work is designed to have both a first-order ( â 1 , λ ≈1,460 nm) and a second-order ( â 2 , λ ≈1,545 nm) optical cavity resonance of high quality factor. Both of these optical cavity modes are dispersively coupled to the same gigahertz-frequency mechanical resonance, depicted in Fig. 1f ( b , ω m /2 π =3.993 GHz, Q m =87 × 10 3 at T≈ 14 K). A tapered optical fibre waveguide, placed in close proximity (~100 nm) to the OMC nanobeam cavity [28] using precision stages, is used to evanescently couple light into and out of the cavity modes. A schematic of the experimental set-up used to characterize the OMC wavelength converter is shown in Fig. 2a . Measurements were performed in vacuum and at low temperature inside a continuous flow cryostat with a cold finger temperature of 9 K (the corresponding sample temperature, as inferred from the thermal bath temperature of the localized mechanical mode of the OMC cavity, is 14 K (ref. 15 )). Initial characterization of the optical cavity modes is performed by scanning the tunable control lasers across a wide bandwidth and recording the transmitted optical intensity through the optical fibre taper waveguide. Such a wavelength scan is shown in Fig. 2b , from which the resonance frequency ( ω 1 /2 π =205.3 THz, ω 2 /2 π =194.1 THz), cavity linewidth ( κ 1 /2 π =520 MHz, κ 2 =1.73 GHz) and waveguide coupling efficiency ( η 1 =0.10, η 2 =0.21) of the two nanobeam cavity modes are determined. 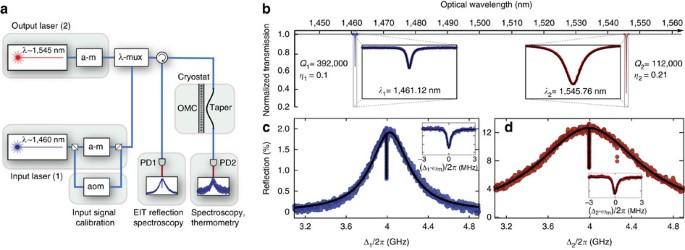Figure 2: Experimental set-up and optical spectroscopy. (a) Two tunable external cavity diode lasers are used as control beams driving the wavelength conversion process. The input (output) control laser is locked as a mechanical frequency red-detuned from the first-order (second-order) cavity mode atλ≈1,460 nm (λ≈1,545 nm). Both control beams can be amplitude modulated (a-m) to perform EIT-like spectroscopy of the cavity modes, or in the case of the input laser, to generate the input sideband signal for the wavelength conversion process. As described in the Methods, an AOM is used to calibrate the input sideband signal. The light from both lasers is combined using a wavelength multiplexer (λ-mux), and then sent into a dimpled optical fibre taper that is coupled to the OMC cavity. The cavity sample is placed in a cryostat to precool it down toT≈14 K. The transmitted light from the cavity is sent to a high-speed photodetector (PD2), which is connected to a spectrum analyser to measure the converted signal on the output laser. The reflected optical signal from the cavity is directed via an optical circulator to a second high-speed photodetector (PD1) to probe the EIT-like spectrum of each cavity mode. (b) Broad wavelength transmission scan showing fibre taper coupling to both the first-order (λ≈1,460 nm) and second-order (λ≈1,545 nm) cavity modes. (c) EIT scan of cavity modeâ1, with inset showing a zoomed-in scan of the transparency window. The solid black lines correspond to fits to a theoretical model allowing extraction of system parameters (κ1,γ,δ1andωm). (d) Corresponding EIT scan of cavity modeâ2. For measurements in both (c,d) the control beam intensities were set such thatγOM,1≈γOM,2>>γi, with detuningsδ1ωmandδ2≈ωm. Figure 2: Experimental set-up and optical spectroscopy. ( a ) Two tunable external cavity diode lasers are used as control beams driving the wavelength conversion process. The input (output) control laser is locked as a mechanical frequency red-detuned from the first-order (second-order) cavity mode at λ≈ 1,460 nm ( λ≈ 1,545 nm). Both control beams can be amplitude modulated (a-m) to perform EIT-like spectroscopy of the cavity modes, or in the case of the input laser, to generate the input sideband signal for the wavelength conversion process. As described in the Methods, an AOM is used to calibrate the input sideband signal. The light from both lasers is combined using a wavelength multiplexer (λ-mux), and then sent into a dimpled optical fibre taper that is coupled to the OMC cavity. The cavity sample is placed in a cryostat to precool it down to T≈ 14 K. The transmitted light from the cavity is sent to a high-speed photodetector (PD2), which is connected to a spectrum analyser to measure the converted signal on the output laser. The reflected optical signal from the cavity is directed via an optical circulator to a second high-speed photodetector (PD1) to probe the EIT-like spectrum of each cavity mode. ( b ) Broad wavelength transmission scan showing fibre taper coupling to both the first-order ( λ ≈1,460 nm) and second-order ( λ ≈1,545 nm) cavity modes. ( c ) EIT scan of cavity mode â 1 , with inset showing a zoomed-in scan of the transparency window. The solid black lines correspond to fits to a theoretical model allowing extraction of system parameters ( κ 1 , γ , δ 1 and ω m ). ( d ) Corresponding EIT scan of cavity mode â 2 . For measurements in both ( c , d ) the control beam intensities were set such that γ OM,1 ≈ γ OM,2 >> γ i , with detunings δ 1 ω m and δ 2 ≈ ω m . Full size image Further characterization of the optomechanical cavity is performed by using the control laser beams in conjunction with a weak sideband probe. With control beams α 1 and α 2 detuned a mechanical frequency to the red of their respective cavity modes ( δ 1,2 = ω m ), a weak sideband signal generated from α 1 is swept across the first-order cavity mode. The resulting reflected sideband signal versus sideband frequency shift Δ 1 is plotted in Fig. 2c , showing the broad cavity resonance along with a narrow central reflection dip (see Fig. 2d inset). The narrow reflection dip, akin to the EIT transparency window in atomic systems, is due to the interference between light coupled directly into the cavity mode and light coupled indirectly through the mechanical mode [24] , [25] . A similar EIT response is shown in Fig. 2d for the second-order cavity mode. Each of the transparency windows occur at Δ k = ω m , with a bandwidth equal to the optically damped mechanical linewidth ( γ = γ i + γ OM,1 + γ OM,2 ). By fitting the optical resonance lineshape and transparency windows to theory, one can also extract the control beam detunings δ k . In what follows, we use this sort of EIT reflection spectroscopy, time-multiplexed in between wavelength conversion measurements, to set and stabilize the frequency of the control beams to δ k = ω m . We note the EIT reflection spectroscopy, though convenient for full characterization and elucidation of the conversion process, is not necessarily performed in a real system application given that both the laser and the cavity resonance have frequency drift, over the measured period of days, that is much smaller than the optical cavity linewidth κ of the devices studied here. Efficiency Coherent wavelength conversion can be thought of as occurring between the input transparency window of â 1 and the output transparency window of â 2 , with the phonon transition mediating the conversion. As shown above, conversion efficiency is theoretically optimized for matched cooperativities of control beam α 1 and α 2 (or equivalently γ OM,1 = γ OM,2 ). Calibration of the optically induced mechanical damping by the control beams can be performed as in the EIT spectroscopy described above, or by measuring the spectral content of the photodetected transmission intensity of â 2 in the absence of any optical input. Such a measurement (see set-up in Fig. 2a and Supplementary Fig. S1 ) measures the mechanical resonator linewidth through the noise spectrum generated by the beating of noise sideband photons generated by thermal motion of the mechanical resonator with the control beam α 2 . Fig. 3a plots the inferred optomechanically induced damping of the mechanical resonator as a function of the power (intracavity photon number, n c ) of control beams α 1 and α 2 , the slope of which gives the zero-point optomechanical coupling for both cavity modes ( g 1 /2 π =960 kHz and g 2 /2 π =430 kHz). 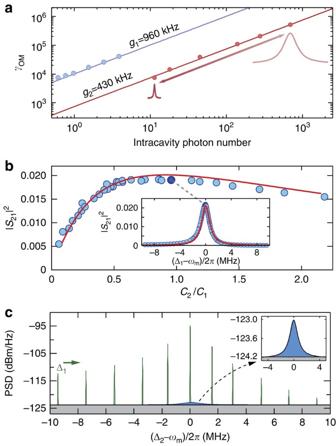Figure 3: Wavelength conversion efficiency and bandwidth. (a) Plot of the optically induced mechanical damping versus control beam intensity (intracavity photon number) for each cavity mode, as measured through the mechanical thermal noise spectrum imprinted on the optical output intensity ofâ2. The calibration curve for cavity modeâ2is performed withα1turned off, whereas the curve for cavity modeâ1is generated with a weakα2such thatγOM,2<<γOM,1for all measured points. (b) End-to-end power conversion efficiency of input signal to output signal for Δ1=0 as a function of the ratio of the cooperativities of the control beams. In this plot, the control beam intensity for the first-order cavity mode is held fixed (withC1≈16), while the intensity of the control beam of the second-order cavity mode is swept fromC2<<C1toC2>C1. The blue circles correspond to measured data points, whereas the solid red line is a theoretical curve using independently measured system parameters. Inset shows the conversion efficiency versus input signal detuning for matched control beamsC1=C2≈16, indicating a conversion bandwidth of ~1.55 MHz. (c) Measured power spectrum of the output optical channel forC1=C2≈16, showing a series (Δ1sweep) of converted input tones (green) sitting on top of a much smaller thermal noise pedestal (blue). Inset shows a zoom-in of the thermal noise pedestal. Figure 3: Wavelength conversion efficiency and bandwidth. ( a ) Plot of the optically induced mechanical damping versus control beam intensity (intracavity photon number) for each cavity mode, as measured through the mechanical thermal noise spectrum imprinted on the optical output intensity of â 2 . The calibration curve for cavity mode â 2 is performed with α 1 turned off, whereas the curve for cavity mode â 1 is generated with a weak α 2 such that γ OM,2 << γ OM,1 for all measured points. ( b ) End-to-end power conversion efficiency of input signal to output signal for Δ 1 =0 as a function of the ratio of the cooperativities of the control beams. In this plot, the control beam intensity for the first-order cavity mode is held fixed (with C 1 ≈16), while the intensity of the control beam of the second-order cavity mode is swept from C 2 << C 1 to C 2 > C 1 . The blue circles correspond to measured data points, whereas the solid red line is a theoretical curve using independently measured system parameters. Inset shows the conversion efficiency versus input signal detuning for matched control beams C 1 = C 2 ≈16, indicating a conversion bandwidth of ~1.55 MHz. ( c ) Measured power spectrum of the output optical channel for C 1 = C 2 ≈16, showing a series (Δ 1 sweep) of converted input tones (green) sitting on top of a much smaller thermal noise pedestal (blue). Inset shows a zoom-in of the thermal noise pedestal. Full size image To quantify the efficiency of the wavelength conversion process, the input cavity control beam α 1 is held fixed at a detuning δ 1 = ω m and a power producing an intracavity photon population of n c,1 =100, corresponding to large cooperativity C 1 ≈16. The input signal, a in , is generated as an upper sideband of α 1 using an electro-optic intensity modulator (the lower sideband is rejected by the wavelength converter as it is detuned to Δ 1 ≈− ω m ). Conversion of the a in sideband to an output signal emanating from cavity mode â 2 is completed by applying control beam α 2 with detuning δ 2 = ω m . The converted output signal sideband emitted from cavity â 2 is beat against the transmitted control beam α 2 on a high-speed photodiode. The amplitude of the input signal tone near resonance with cavity mode â 1 is calibrated using a second reference signal generated through acousto-optic modulation of α 1 , whereas the amplitude of the output signal sideband is inferred from calibration of the control beam intracavity number n c,2 and the optical transmission and detection chain (see Fig. 2a and Supplementary Fig. S1 ). Figure 3b plots the resulting power conversion efficiency, given by the magnitude squared of equation (2), versus the ratio of C 2 / C 1 as the power of control beam α 2 is varied and for an input signal exactly resonant with cavity mode â 1 (Δ 1 = ω m ). The power conversion is referred directly to the input and output of the optomechanical cavity (that is, not including additional losses in the optical link). The solid red line shows the theoretical model for the conversion efficiency using the independently measured system parameters, and taking into account power-dependent effects on the optical losses in the silicon cavity modes (see Methods). Good correspondence is seen between the measured data and theory, with a maximum of the conversion occurring at C 1 ≈ C 2 as expected from the matching condition. Bandwidth The bandwidth of the wavelength conversion process is also probed, using matched conditions ( C 1 = C 2 ≈16), and as above, with control beam detunings δ k = ω m . The modulation frequency generating a in is now varied from (Δ 1 − ω m )/2 π =−10 MHz to +10 MHz, sweeping the narrow-band input sideband signal across the transparency window of cavity mode â 1 . The corresponding measured output signal frequency shift follows that of the input signal (Δ 2 =Δ 1 ), with the resulting power conversion efficiency plotted in the inset of Fig. 3b . A peak efficiency, measured from the input to the output port at the optomechanical cavity system, is η =2.2%, corresponding to an internal conversion efficiency of η max,int =93%. Fitting the results to a Lorentzian as in equation (1), we find the conversion bandwidth to be 1.55 MHz, equal to the optically damped mechanical linewidth of the mechanical resonance, γ /2 π . Noise The spectrum of the converted output signal for a series of signal frequencies Δ 1 are shown in Fig. 3c . As can be seen from this plot and the zoomed-in inset, the narrow-band-converted photons sit atop a noise pedestal of bandwidth corresponding to the damped mechanical resonator. This noise is quantified by the added noise quanta number component of equation (2). As shown in the Supplementary Methods , under matched conditions the theoretical added noise is, where the first term arises owing to thermal noise of the cooled and damped mechanical resonator, and the last two terms are quantum noise resulting from the spontaneous scattering of the control beams (quantum back-action noise [29] ). These sources of noise are independent and uncorrelated and as such, add together incoherently. 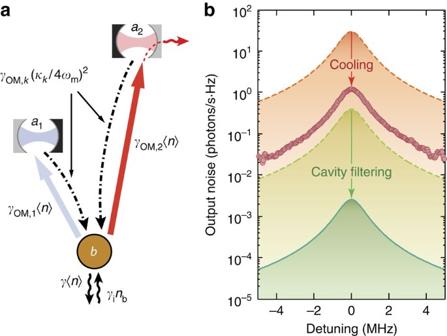Figure 4: Output noise. (a) Schematic showing the relevant input noise terms contributing to the total noise at the output. The rates of ‘noisy’ phonon generation areγinbowing to the thermal bath andγOM,(1,2)(κ(1,2)/4ωm)2owing to spontaneous Stokes scattering from the two control beams. Cooling of the mechanical mode is also performed by the control beams, resulting in a theoretically cooled phonon occupancy of ‹n›=(1/γ) × (γinb+ΣjγOM,j(κj/4ωm)2). The output noise power is proportional to the output cavity cooling rate,γOM,2‹n›. (b) Output noise power spectral density. The measured noise data (red circles) is shown along with several theoretical noise curves. The dashed red curve is the corresponding output noise power in the absence of control beam cooling. The solid (dashed) green curve is the output noise power owing to spontaneous Stokes scattering in the presence (absence) of cavity filtering. Figure 4a pictorially indicates the various cooling, heating and spontaneous scattering mechanisms that lead to the output noise of â 2 . A plot showing the measured output noise spectral density, calibrated in units of photon number, is given in Fig. 4b for the optimal conversion efficiency of Fig. 3b . From the peak of the output noise spectral density (= η 1 η 2 n added ) in this plot, the added noise referred to the input of â 1 is estimated to be n added ≈60 quanta. The corresponding internal added noise (for η =1) is only n added ≈6, predominantly owing to the cooled phonon occupation of the mechanical resonator (‹ n ›≈3). Owing to the strong filtering provided by the high- Q cavities ( κ k / ω m <<1), the quantum back-action noise contributes an insignificant 4 × 10 −2 (4 × 10 −3 ) added input (internal) noise photons. The effectiveness of noise reduction in the optomechanical cavity system is highlighted in Fig. 4b by showing the estimated thermal output noise in the absence of sideband cooling by the control beams (dashed red curve) and the quantum back-action noise in the absence of cavity filtering (green dashed curve). Figure 4: Output noise. ( a ) Schematic showing the relevant input noise terms contributing to the total noise at the output. The rates of ‘noisy’ phonon generation are γ i n b owing to the thermal bath and γ OM,(1,2) ( κ (1,2) /4 ω m ) 2 owing to spontaneous Stokes scattering from the two control beams. Cooling of the mechanical mode is also performed by the control beams, resulting in a theoretically cooled phonon occupancy of ‹ n ›=(1/ γ ) × ( γ i n b +Σ j γ OM, j ( κ j /4 ω m ) 2 ). The output noise power is proportional to the output cavity cooling rate, γ OM,2 ‹ n ›. ( b ) Output noise power spectral density. The measured noise data (red circles) is shown along with several theoretical noise curves. The dashed red curve is the corresponding output noise power in the absence of control beam cooling. The solid (dashed) green curve is the output noise power owing to spontaneous Stokes scattering in the presence (absence) of cavity filtering. Full size image Although the demonstrated wavelength conversion in this work represents an important proof of principle, there are still considerable practical challenges to utilizing such cavity-optomechanical devices for classical or quantum wavelength translation [2] , [9] . With a thermal phonon occupancy ‹ n ›≤ η 1 /2 required for single-photon conversion at unity signal-to-noise, a primary concern for quantum networking [1] is the thermal energy stored in the mechanical resonator. Although resolved sideband cooling of nanomechanical resonators to occupancies below one has recently been demonstrated [14] , [15] , this relation emphasizes the additional need for efficient cavity coupling. For chip-scale photonic devices similar to the one presented here, the technology already exists for efficient optical connectivity, with optical fibre-to-chip coupling of ~95% (ref. 30 ) and waveguide-to-cavity coupling efficiency of η 1 0.999 having been realized [31] . Further reduction in the output noise may also be realized by simply reducing the temperature of operation; for the 4 GHz phonon frequency of the device in this study, n b 10 −3 for a bath temperature of T ~10 mK realizable in a helium dilution refrigerator. Integration of cavity-optomechanical devices into milliKelvin experiments is particularly relevant for superconducting quantum circuits, which themselves have already been strongly coupled to mechanical resonators [32] . Addition of an optical cavity coupled directly, or via an additional acoustic waveguide, to the same mechanical resonator would provide a microwave-to-optical quantum interface [17] , [19] similar to the optical-to-optical interface shown here. In the case of solid-state qubits with optical transitions far from the telecommunication bands, such as the nitrogen-vacancy electron spin in diamond [33] , the radiation pressure nonlinearity of cavity optomechanics could be substituted for intrinsic materials nonlinearities in proposed cavity-based schemes for single-photon wavelength conversion and pulse shaping [34] . Owing to the excellent mechanical properties of diamond and recent advancements in thin-film diamond photonics [35] , a cavity-optomechanical wavelength converter could be fabricated around an nitrogen-vacancy qubit from the same diamond host. During the preparation of this manuscript, a similar work appeared on the arXiv [36] . Generation and conversion of the input signal We begin by considering the input signal to the first optical cavity mode. This signal is generated by weakly modulating the α 1 control beam (represented by amplitude A 1 ) at a frequency Δ 1 using an electro-optic modulator (EOM) producing where β 1 is the modulation index of the input signal and φ accounts for any phase difference between the sidebands ( φ =0 if there is pure amplitude modulation). The input sideband at frequency ω l,1 +Δ 1 is nearly resonant with the first cavity mode at ω 1 , whereas the lower frequency sideband at ω l,1 −Δ 1 is detuned by ~−2 ω m . As such, only the upper frequency sideband is resonant with the transparency window of the first cavity mode, and only this sideband is converted by the OMC cavity into a sideband at the second, output cavity mode â 2 . The converted sideband is generated from the control laser beam α 2 of the second cavity mode with frequency ω l,2 +Δ 1 . Thus, the output field amplitude near the frequency of the second control laser beam (amplitude A 2 ) is, ignoring φ , The power measured by a photodetector from the optical signal eminating from the output cavity mode is proportional to We thus define β 2 =| s 21 (Δ 1 )| β 1 A 1 /4 A 2 as the modulation index of the output signal, By careful calibration of β 1 and β 2 , and measurement of the control beam power the conversion scattering matrix element can be determined: Calibration of the input signal The appearance of φ in equation (5), along with its sensitivity to effects such as chromatic dispersion in the optical fibre and components, make calibration of β 1 more challenging owing to interference between the upper and lower frequency sidebands. Direct photodetection of the optical input signal results in a φ -dependent measured beat signal between the carrier and the two sidebands. To bypass this problem, we generate an additional single sideband using an acousto-optic modulator (AOM), and beat it against each of the input optical sidebands. This is accomplished by splitting off a portion of the optical input signal before creating the EOM sidebands, and frequency shifting it by Δ AOM (see Supplementary Fig. S1 ). This AOM-shifted signal is then recombined with the main input signal, giving an overall signal equal to where A 3 is the field amplitude of the signal split off from the input signal before the EOM. The total photodetected signal is then given by From this equation, we see that the optical power at the detector consists of components at zero frequency (DC) as well as four modulated tones (see Supplementary Fig. S2 ). By taking the ratio of the tone at Δ AOM and Δ 1 −Δ AOM , the value of β 1 can be accurately determined, independent of φ . Note that in order to determine β 2 no such additional calibration signal is required. The filtering properties of the input and output cavities results in a single output sideband, with no phase dependence of the photodetected intensity spectrum. In this case, careful optical and electronic calibration of the measured output cavity ( â 2 ) optical transmission intensity, similar to that described in the Supplementary Information of [15] , provides an accurate estimate of β 2 and the wavelength-converted signal strength. Power-dependent optical cavity loss To model the wavelength conversion process, all of the optical cavity mode and mechanical resonator parameters entering into equation 1 must be independently determined. Most of these parameters are measured as described in the main text; however, additional measurements were performed to determine the power-dependent optical cavity loss in the silicon OMC device. Owing to two-photon absorption in silicon, the parasitic optical cavity loss of both cavity modes is not static, but rather depends upon both control beam powers. This effect is particularly acute for the higher Q -factor first-order cavity mode ( â 1 ), where in Supplementary Fig. S3a we plot the normalized on-resonant optical transmission ( T 0,1 ) of the first-order cavity mode versus the power (as represented by the intracavity photon population, n c,2 ) of control beam α 2 feeding the second-order cavity mode. The steady rise in the on-resonance transmission versus n c,2 is attributable to the increased optical absorption loss stemming from free carriers generated by two-photon absorption of the control beam α 2 . The corresponding change in coupling efficiency, η 1 ≡ κ e,1 /2 κ 1 , is shown on the right-side axis of Supplementary Fig. S3a . Neglecting the effects of nonlinear optical absorption and free carriers on the intrinsic optical quality factor of â 1 leads to a theoretical model of conversion efficiency denoted by the dashed black line in Supplementary Fig. S3b . Taking into account the nonlinear optical loss measured in Supplementary Fig. S3a leads to the theoretical conversion efficiency denoted by the solid red line, showing much better correspondence with the data (the solid red line is the model fit shown in the main text). The effect of two-photon absorption and free-carrier absorption is much smaller on the second-order cavity mode ( â 2 ) owing to its already lower optical Q -factor, and we neglect it here. The control-beam-generated free carriers also affect the intrinsic mechanical quality factor ( γ i ) as was shown in [15] ; however, this effect is small for the control beam powers studied here (the efficiency curve of Supplementary Fig. S3b is also not modified as we plot it versus the ratio of cooperativities for which γ i cancels out). How to cite this article: Hill, J.T. et al . Coherent optical wavelength conversion via cavity optomechanics. Nat. Commun. 3:1196 doi: 10.1038/ncomms2201 (2012).